Robust quantum metrological schemes based on protection of quantum Fisher information Fragile quantum features such as entanglement are employed to improve the precision of parameter estimation and as a consequence the quantum gain becomes vulnerable to noise. As an established tool to subdue noise, quantum error correction is unfortunately overprotective because the quantum enhancement can still be achieved even if the states are irrecoverably affected, provided that the quantum Fisher information, which sets the ultimate limit to the precision of metrological schemes, is preserved and attained. Here we develop a theory of robust metrological schemes that preserve the quantum Fisher information instead of the quantum states themselves against noise. After deriving a minimal set of testable conditions on this kind of robustness, we construct a family of 2 t +1 qubits metrological schemes being immune to t -qubit errors after the signal sensing. In comparison, at least five qubits are required for correcting arbitrary 1-qubit errors in standard quantum error correction. In quantum metrology, delicate and fragile quantum features are being used to enhance the sensitivity of experimental apparatus, for example, non-classical probe states were used for the high sensitivity of optical interferometer and atomic spectroscopy [1] , [2] , [3] , [4] , [5] , [6] , [7] , [8] . However, the quantum enhancement for the sensitivity may be subdued by the presence of ubiquitous and inevitable noise [9] , [10] , [11] , [12] , [13] , [14] , [15] , [16] , [17] , [18] , [19] , [20] , [21] , [22] , [23] , [24] , [25] , [26] . Therefore, it is of utmost significance to investigate the robustness of the optimal strategies for the high sensitivity against noise. Most recently, quantum error correction (QEC) was employed in quantum metrology [27] , [28] , [29] , [30] to overcome noise problem, whereby protecting the quantum states, on which a signal parameter is imprinted, the measurement precision for that parameter is protected. This is no wonder because the standard QEC was originally designed for protecting all the information encoded in quantum states, that is, the logical states in the universal quantum computation, against the noise [31] , [32] , [33] , [34] , [35] , [36] , [37] . In quantum metrology, however, what matters essentially is the distinguishability about the signal parameter that is sensed by quantum systems and encoded in quantum states. According to the quantum estimation theory [38] , [39] , [40] , [41] , [42] , this distinguishability is measured by quantum Fisher information (QFI). Therefore, preserving the QFI of a given family of states against noise is sufficient for quantum metrological schemes to work under noisy environment. Since the QFI represents only partial information encoded in quantum states, the use of the QEC for quantum states is obviously overprotective, which leads to unnecessary waste of resources. Our main goal is to establish a variant theory of QEC designed for quantum metrology, namely, robust quantum metrological schemes, by taking the QFI instead of the fidelity of quantum states as the figure of merit. In this paper, we show that analogous to QEC for quantum states the errors can also be digitalized so that we can construct a robust metrological scheme, in which the QFI is preserved under an entire class of unknown noisy processes rather than a specific one. Furthermore, we derive the necessary and sufficient testable conditions on preserving QFI, and construct the optimal measurements extracting the maximal distinguishability about the signal parameter in the presence of noise. Our testable conditions describe the minimal requirements for the robustness of a parameter estimation scheme against noise, and can be used to identify the errors to which the QFI is immune. As an example, we construct a family of metrological scheme on 2 t +1 physical qubits to protect the QFI against arbitrary errors on no more than t physical qubits after the signal sensing. Quantum parameter estimation theory A standard quantum metrological scheme to detect and estimate a signal parameter θ can be depicted by the following sensing transformation: with H being a known Hermitian operator and ρ the probe state. The value of the parameter is estimated through the classical data processing on the measurement outcomes obtained by repeating experiments in ρ θ . From estimation theory [38] , [39] , [40] , the regularized root mean squared error of the estimator is limited by the Cramér–Rao bound where ν is the number of repetitions of the experiments, and is the (classical) Fisher information extracted by the measurement { M x } with p θ ( x ):=Tr( M x ρ θ ) being the probabilities of obtaining outcomes x . Here M x are positive operators satisfying with 1 being the identity operator. The maximal Fisher information over all possible measurements is given by the so-called QFI where the symmetric logarithmic derivative (SLD) operator L θ is defined as the Hermitian operator satisfying with {·,·} being the anti-commutator [38] , [39] , [40] , [41] , [42] . More importantly, the Cramér–Rao bound is asymptotically achieved [38] , [39] , therefore, QFI can be considered as a measure on the distinguishability about the parameter in quantum states. An optimal strategy of the quantum parameter estimation comprises the probe state maximizing the QFI and the measurement attaining the maximal Fisher information. Taking appropriate entangled states as the probe states, a quantum metrological scheme may achieve the Heisenberg scaling of precision 1/ N , where N is the number of resources employed in the experiment, for example, the number of probes [6] , [7] , [8] . This is a considerable improvement over the standard quantum limit . Nevertheless, those entanglement-enhanced strategies that are optimal for the noiseless systems easily lose the quantum gain for the noisy systems [9] , [11] , [12] , [14] , [15] , [16] , [17] , [18] , [19] , [20] , [21] , [22] , [23] , [24] , [25] , [26] . Parameter estimation in noisy cases We now turn to the question of the optimal strategy in noisy cases. We assume that the noise can be deferred until after the sensing transformation, that is, states to be measured are where denotes a noisy channel with Kraus operators { E j }. We emphasize that this noise model is applicable to the noise that commutes with the generator of the sensing transformation, occurs during the transmission or storage in the interval between the sensing and the measurement, or is induced by the measurement imperfection. This noise model can also be considered as an approximation when the sensing time is short [27] , [28] . A general entanglement-enhanced metrology scenario of this type is depicted in Fig. 1a . At first glance, the optimal strategy for such noisy cases might be established by seeking the optimal probe states maximizing the QFI of and the corresponding optimal measurements. Technically, this straightforward optimization needs to diagonalize the parametric family of states , which is often formidable and even impossible without the details of the noise. Therefore, the optimal strategies obtained in this way are very restricted. 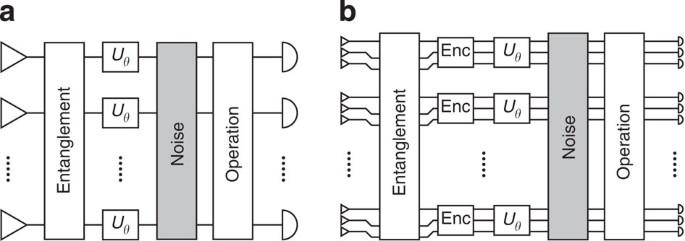Figure 1: Abstract models for quantum parameter estimation. (a) Set-up for entanglement-enhanced metrology with noise being assumed after the sensing transformation, wherenis the number of the qubits. (b) Heisenberg-limited metrological scheme with the QEC protection. The entangling operation (labelled with ‘Entanglement’ in the figure) acts only on the first qubit (thick line) in each block, and produce the GHZ state. The encoders (labelled with ‘Enc’) encode the first qubit in each block into a phase-flip code. The sensing transformationUθis a logical phase-shift operation on each phase-flip code space. Here we note that the ‘Entanglement’ operation plays a dual role: on one hand, it supplies the Heisenberg scaling of the QFI, and on the other hand, it supplies a higher level of bit-flip code in addition to the phase-flip code. Figure 1: Abstract models for quantum parameter estimation. ( a ) Set-up for entanglement-enhanced metrology with noise being assumed after the sensing transformation , where n is the number of the qubits. ( b ) Heisenberg-limited metrological scheme with the QEC protection. The entangling operation (labelled with ‘Entanglement’ in the figure) acts only on the first qubit (thick line) in each block, and produce the GHZ state. The encoders (labelled with ‘Enc’) encode the first qubit in each block into a phase-flip code. The sensing transformation U θ is a logical phase-shift operation on each phase-flip code space. Here we note that the ‘Entanglement’ operation plays a dual role: on one hand, it supplies the Heisenberg scaling of the QFI, and on the other hand, it supplies a higher level of bit-flip code in addition to the phase-flip code. Full size image On the basis of the above considerations, protecting the involved parametric family of states with quantum error-correcting codes [31] , [32] , [33] , [34] , [35] , which are applicable for the whole class of noisy channels with the Kraus operators being arbitrary linear combinations of the correctable error elements, is a good candidate of a robust strategy for quantum metrology [27] , [28] , [29] , [30] . However, QEC is overprotective because the measurement precision remains the same as long as the QFI is preserved and attained, even if the quantum states might be affected by some uncorrectable errors. Here we shall develop a theory of QEC specialized for metrology: on the one hand, our theory aims at preserving the QFI instead of all the information encoded in states, which ensures that our robust quantum metrological schemes are not overprotective; on the other hand, our specialized theory also possesses the great advantage of the standard QEC that the errors can be digitalized for the preservation and attainment of QFI, which is our first main result: Theorem 1: the QFI of ρ θ is preserved under a known channel with Kraus operators { E j } if and only if with being the SLD operator for . If the QFI of ρ θ is preserved under a known noisy channel , then it is preserved under all noisy channels whose Kraus operators are arbitrary linear combinations of { E j }, with the optimal measurement being the eigenstates of . We split the proof of Theorem 1 into three parts. First, we prove in the Methods that equation (1) is the necessary and sufficient condition on QFI preserving under a known noisy channel. Second, for an arbitrary noisy channel with Kraus operators being unknown linear combinations of { E j }, we note that equation (4) still holds with E j being replaced by K j , therefore, the QFI is preserved under the unknown noisy channel . Third, it is known that the complete set of the eigenstates of the SLD operator is the optimal measurement basis attaining the maximal Fisher information [40] . Through equation (4), the SLD operator for can be readily checked to be also the SLD operator for . Therefore, the measurement with respect to eigenstates of is also optimal for . Remarkably, if the measurement basis is fixed, then a recovery operation is demanded to transform the basis of the optimal measurement to the fixed one; otherwise, we only need to perform the optimal measurement for noisy states, and no recovery operation is demanded. Theorem 1 can be understood in a geometric way. On the manifold of pure states, there is a Riemannian metric known as the Fubini–Study metric [43] , [44] . Along the parametric states , a line element is given by with being the covariant derivative vector. This geometric metric is connected to parameter estimation theory in twofold: on one hand, the QFI is given by ; on the other hand, the SLD operator is a Hermitian representation of the covariant derivative as , and the projective measurement with respect to eigenstates of attains the maximal Fisher information. In Fig. 2 , we show that how the conditions on the preservation of QFI can be intuitively understood in this geometric picture. 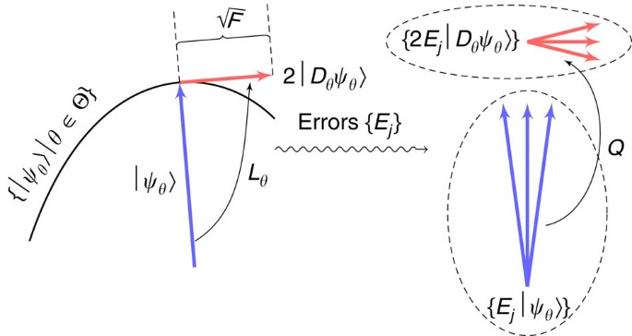Figure 2: Geometrical picture for preserving QFI. The QFIFofequals to the square of the Euclidean length ofin terms of the Fubini–Study metric on the manifold of pure states, whereis the covariant derivative. For pure states, the symmetric logarithmic derivative operatorLθis a Hermitian representation of the covariant derivative as, and the projective measurement with respect to eigenstates ofLθattains the maximal Fisher information. Under a set {Ej} of errors, parametric state vectors are transformed into, while covariant derivative vectors into. The QFI is preserved under the errors if and only if there exists a Hermitian operatorQtransforming all the erroneous state vectors to the corresponding erroneous covariant derivative vectors, that is,for allj; this operatorQactually is the symmetric logarithmic derivative operator for all the noisy states under the errors (see the Methods section). The projective measurement with respect to eigenstates ofQattains the maximal Fisher information in noisy states. Figure 2: Geometrical picture for preserving QFI. The QFI F of equals to the square of the Euclidean length of in terms of the Fubini–Study metric on the manifold of pure states, where is the covariant derivative. For pure states, the symmetric logarithmic derivative operator L θ is a Hermitian representation of the covariant derivative as , and the projective measurement with respect to eigenstates of L θ attains the maximal Fisher information. Under a set { E j } of errors, parametric state vectors are transformed into , while covariant derivative vectors into . The QFI is preserved under the errors if and only if there exists a Hermitian operator Q transforming all the erroneous state vectors to the corresponding erroneous covariant derivative vectors, that is, for all j ; this operator Q actually is the symmetric logarithmic derivative operator for all the noisy states under the errors (see the Methods section). The projective measurement with respect to eigenstates of Q attains the maximal Fisher information in noisy states. Full size image Theorem 1 concerns the robustness of quantum parameter estimation with respect to noise. It suggests that there might be a probe state that does not maximize the QFI under a specific noisy channel but ensures the QFI to be preserved and attained under an entire class of noisy channels. The necessary and sufficient condition (4) on preserving the QFI against a set of errors needs the SLD operator for the corresponding noisy state . Our second main result is the testable conditions on preserving QFI without referring to the SLD operators of the noisy state. These testable conditions are useful for finding good probe states for certain errors, or identifying those errors to which the QFI with certain probe state is immune. Theorem 2: the QFI of is preserved under a set { E j } of errors, if and only if (i) for all j and k , and (ii) for some α j ∈ infers . For mixed state ρ θ , the QFI is preserved if and only if the above two conditions hold for all the states in the range of ρ θ . The proof is sketched in the Methods (a full version is deferred to the Supplementary Note 1 ). For a unitarily parameterized family of pure states, , by noting with , we simplify the two testable conditions into the following: (i) for all j and k and (ii) for some α j ∈ infers . The testable conditions describe the minimal requirements for the robustness of a parameter estimation scheme against noise, and are looser than that of QEC for the parametric family of states. Recall that a set { E j } of errors is correctable for a code space if and only if are satisfied for all j , k and all pairs of orthonormal state vectors and in the code space [35] . Let us choose and H to be in a standard quantum error-correcting code so that and are two orthonormal states in the coding subspace. In such case, the first and second testable conditions are implied by the first and second equalities in equation (7), respectively. Henceforth, we simply say that ρ θ is a robust metrological scheme with respect to a set { E j } of errors if the QFI of ρ θ is preserved under { E j }. We show below that concrete robust metrological schemes can be easily constructed based on the stabilizer formalism [34] . A stabilizer code is the joint +1 eigenspace of the stabilizer group S , which is an Abelian subgroup of the n -qubit Pauli group, that is, for all S i ∈ S and all . A set { E j } of Pauli errors— E j are also elements of the n -qubit Pauli group—are correctable for this stabilizer code, if each is either in the stabilizer group, or detectable, that is, anticommutes with at least one element of the stabilizer group [34] . Theorem 3: in a metrological scheme where the probe state is taken from the coding subspace of a stabilizer code capable of correcting errors { E j } and [ H , S ]=0, the QFI is also immune to the errors , where is a Pauli error that commutes with S while anticommutes with with P being the projection onto . If the coding subspace is two dimensional, then the optimal measurement is the joint measurement of S and . The proof is sketched in the Methods (see Supplementary Note 1 for a full proof). Theorem 3 can be easily used to identify the QFI-immune error set for a given scheme. As an example, we consider a system composed of n =2 t +1 qubits that are labelled with the index set I ={1, 2, …, n }. Let us denote X i , Y i and Z i the tensor products of the Pauli matrices X , Y and Z on the i th qubit and identity operators on other qubits, respectively, and with for O = X , Y and Z . Let be the two-dimensional subspace stabilized by { X α || α |=even}, which is exactly the coding subspace of a stabilizer code capable of correcting all t -qubit phase-flip errors { Z α } with | α |≤ t . For any state such that , the metrological scheme preserves QFI against all t -qubit phase-flip errors plus errors of type { Z α X I }, which include essentially arbitrary error on no more than t qubits, that is, those whose error operators have nontrivial effects on no more than t qubits. That is to say, in terms of QFI, the t -qubit phase-flip codes can be used to protect a metrological scheme from arbitrary t -qubit errors occurring after the signal sensing. In comparison, at least five physical qubits are required in a standard quantum error-correcting code to correct arbitrary single-qubit error, while our scheme requires only three physical qubits. This is one of the advantages brought in by considering the preservation of QFI instead of the protection of quantum states. The maximal Fisher information is attained by the joint measurement of the stabilizers of and X I , that is, all the observables { X i | j ∈ I } without any recovery operation. Entanglement-enhanced metrology Beating the standard quantum limit by quantum entanglement is one of the most fascinating aspects of the quantum-enhanced metrology [6] , [7] , [8] . A canonical example is utilizing the m -qubit Greenberger–Horne–Zeilinger (GHZ) state as the probe state for the parallel samplings of a unitary sensing transformation, wherein QFI scales quadratically with m —the Heisenberg scaling. Replacing the noisy individual systems in the entangled state by logical ones makes the resulting scheme robust to correctable errors [27] . Here we show that the entanglement, besides helps to beat the standard quantum limit, also supplies a higher level of quantum error-correcting code. Let us consider a metrological scheme whose parametric family of states read where are the logical Pauli Z operators on the i th block, and and are the logical basis states. Let be the stabilizer group of the n -qubit phase-flip code for the i th qubit in the original scheme. Further, assume that m and n =2 t +1 are odd. This scheme is robust against to three kinds of errors occurring after the signal sensing. First, less than or equal to t phase-flip errors are correctable by phase-flip code in each block. Second, the states given by equation (8) are in a subspace stabilized by , which is a bit-flip code capable of correcting no more than ( m −1)/2 logical bit-flip errors in the blocks. Since every single-qubit bit-flip error on the codewords of the phase-flip code in each block is equivalent to a logical bit-flip error on the block, less than or equal to ( m −1)/2 physical bit-flip errors are correctable. Third, for more than ( m −1)/2 bit-flip errors, the parametric family of states cannot be recovered but the QFI is still preserved. Moreover, the joint measurement of all the stabilizers and of the stabilizer code together with attain the maximal Fisher information. In ref. 27 , Dür et al . proposed the same metrological scheme as equation (8) but only the protective capability of the error-correcting codes in each block was explored; we note that the GHZ state itself provides a higher-level bit-flip code and find some uncorrectable errors that are harmless to QFI. Noise during the signal accumulation The above results still hold for the noise during the signal accumulation if the generator of the noise commutes with that of the signal accumulation. A simple case of this kind is that the error operators E j commute with the generating operator H of the signal accumulation; but in such a case, our method is equivalent to the protection of quantum states [27] as the additional errors given by theorem 3 do not commute with H . However, the errors that can be deferred after the signal accumulation are not restricted in this case. Therefore, our method still has potential advantages over the protection of quantum states for the deferrable noise. Let us consider a quantum system that evolves as where ω is the signal parameter to be sensed and estimated, the superoperators and are the generators of the signal accumulation and the noise, respectively. Usually, so that for the noiseless case the signal accumulation is unitary. The noise can be deferred after the signal accumulation if the superoperator commutes with , so that the total evolution is . This does not imply that the Kraus operators for commute with the operator H . For example, let us consider the phase accumulation of an atom under spontaneous emission, where H = Z and with σ _=( X − iY )/2. The Kraus operators for are given by and with η = e − γt . It can be shown that commutes with , nevertheless [ E 2 , H ]≠0. Physical example Here we give a physical example to quantitatively analyse the performance of robust metrological schemes with the QFI protection. Let us consider the frequency estimation of atoms with uncorrelated parallel and transverse dephasing. The atoms are modelled by qubits whose evolution is still in the form of equation (9). The noise is described by , where γ x and γ z are the strengths of the noise, , and with N being the total number of qubits. The qubits are divided into blocks. The probe state is the logical GHZ states with respect to n -qubit phase-flip code in each block, and the generating operator of the signal accumulation is given by . This scheme was first proposed by Dür et al . [27] to subdue only the parallel dephasing. When n =1, this scheme is reduced to the ordinary one of using the raw GHZ probe state and independent signal accumulation [6] . Note that commutes with both and . For short measurement times such that and Nω 2 t 2 <<1, by approximation of Trotter expansion, it can be shown that . Note that for a = x , z with and , where . In the case of the raw GHZ state scenario (that is, n =1), we obtain the exact result of the QFI about ω as where (See Supplementary Note 2 for the detailed calculations). When γ x =0, we have , which is consistent with the result of ref. 9 . When γ z =0, we have F [ ρ ( t )]= N 2 t 2 , which is consistent with theorem 3 as the QFI is totally preserved if there are only bit-flip errors. Note that this is not explicit if we only consider the protection of quantum states. Moreover, as long as p z is small such that (1−2 p z ) N is close to 1, the QFI of the noisy states is close to N 2 t 2 and insensitive to p x . Therefore, the phase-flip code is enough to protect the QFI against the parallel and transversal dephasing in such a situation. The logical GHZ state scenario, where n is an odd number greater than one, can be recast into the raw GHZ state scenario by noting that only logical errors remain after the error correction in each block. Since less than or equal to ( n −1)/2 phase-flip errors are corrected, the probability of the logical phase-flip error is suppressed to , see ref. 27 . Note that each single-qubit bit-flip error is equivalent to a logical bit-flip error on that block. The probability of the logical bit-flip error is . Then, the QFI of the noisy states in the logical GHZ state scenario can also be given through equations (10) and (11) via substituting p x , p z and N by , and , respectively. Note that for 0< p x <1/2, which means that the bit-flip errors are amplified. However, as long as the phase-flip errors are sufficiently suppressed, the bit-flip errors in the GHZ state scenario are almost harmless to QFI. For instance, it is shown in Fig. 3 that in the raw GHZ state scenario the quantum Cramér–Rao bound rises when the destructive effect of the noise on the QFI is dominant over the gain of the signal accumulation, whereas the use of the error correction can suppress the phase-flip errors so that the quantum states can gain more QFI by the signal accumulation process for a long time even in the presence of the bit-flip errors. In Fig. 4 , we show that using the phase-flip QEC code the quantum Cramér–Rao bound has a Heisenberg scaling with a constant factor, that is, . Note that here the size n of the block is a fixed small integer, for example, n =3 for the three-qubit phase-flip code in each block. Therefore, when N becomes large, n / N will be much smaller than the standard quantum limit . In this comparison, the resources are measured by the total number of the physical qubits used. However, it should be noted that the signal accumulation processes are different in the two scenarios. 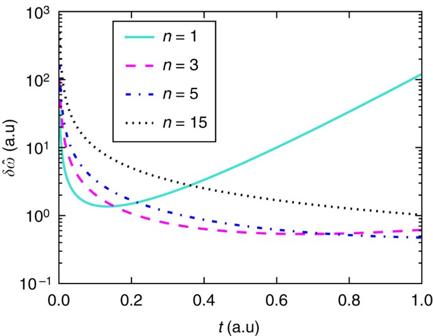Figure 3: Quantum Cramér–Rao bounds of a single-shot measurement. The estimation error, represented by the vertical axis, is bounded from below by the quantum Cramér–Rao bounds (the curves in the figure). The horizontal axis represents the time of the signal accumulation process. Here the total number of qubits isN=15, which is divided into blocks of sizen=1, 3, 5 and 15. Each block is protected by ann-qubit phase-flip code. The probe state is the logical GHZ state, and the sensing transformation is the independent logical phase accumulation. The figure is plotted atω=0.001,γx=0.001 andγz=0.5. Figure 3: Quantum Cramér–Rao bounds of a single-shot measurement. The estimation error , represented by the vertical axis, is bounded from below by the quantum Cramér–Rao bounds (the curves in the figure). The horizontal axis represents the time of the signal accumulation process. Here the total number of qubits is N =15, which is divided into blocks of size n =1, 3, 5 and 15. Each block is protected by an n -qubit phase-flip code. The probe state is the logical GHZ state, and the sensing transformation is the independent logical phase accumulation. The figure is plotted at ω =0.001, γ x =0.001 and γ z =0.5. 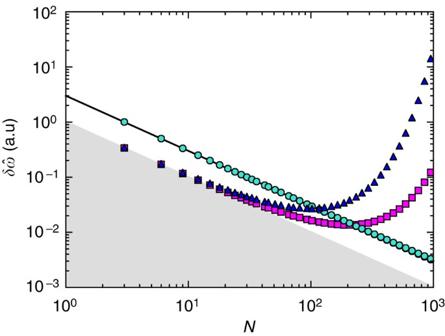Figure 4: Quantum Cramér–Rao bounds as a function of the total number of qubits. The grey region denotes where the uncertainty is below the Heisenberg limit 1/N. In the scenario of using the raw GHZ states and the raw phase accumulation, the quantum Cramér–Rao bounds cannot follow the Heisenberg scale whenNis large, see the magenta square markers for the first kind of noise withγx=5 × 10−4andγz=5 × 10−3, and the blue triangle markers for the second kind of noise withγx=10−3andγz=10−2. In the scenario of using the logical GHZ states and the logical phase accumulation with the three-qubit phase-flip code in each block, the quantum Cramér–Rao bounds for the first and second kinds of noise are so close that they are visually indistinguishable in the figure (denoted by turquoise circle marker), which reflects the robustness of the scheme. Furthermore, in the logical scenario, the quantum Cramér–Rao bounds follow well the Heisenberg scale of 3/N(black solid line). The figure is plotted atω=0.001 andt=1. Full size image Figure 4: Quantum Cramér–Rao bounds as a function of the total number of qubits. The grey region denotes where the uncertainty is below the Heisenberg limit 1/ N . In the scenario of using the raw GHZ states and the raw phase accumulation, the quantum Cramér–Rao bounds cannot follow the Heisenberg scale when N is large, see the magenta square markers for the first kind of noise with γ x =5 × 10 −4 and γ z =5 × 10 −3 , and the blue triangle markers for the second kind of noise with γ x =10 −3 and γ z =10 −2 . In the scenario of using the logical GHZ states and the logical phase accumulation with the three-qubit phase-flip code in each block, the quantum Cramér–Rao bounds for the first and second kinds of noise are so close that they are visually indistinguishable in the figure (denoted by turquoise circle marker), which reflects the robustness of the scheme. Furthermore, in the logical scenario, the quantum Cramér–Rao bounds follow well the Heisenberg scale of 3/ N (black solid line). The figure is plotted at ω =0.001 and t =1. Full size image The scenario considered in this work assumes a model where the noise occurs after the signal sensing. This coincides with analogue communication over noisy quantum channels [45] , where analogue signals are encoded in quantum states, transmitted over a noisy quantum channel and estimated by the receivers. The assumed model is also applicable for the sensing-stage noise whose generator is commuting with that of the signal sensing. Some known examples belonging to this class include the depolarization, the dephasing and the spontaneous emission [11] in the two-level systems with the signal sensing generated by the Pauli Z matrix, and the photon loss [16] and the phase diffusion [25] in the optical fields with the signal sensing generated by the photon number operator. For realistic instruments where the noise may be very complicated, our method can be applied together with other technologies such as dynamical decoupling [29] . In summary, we have established a theory of error correction designed for quantum metrology in the context of quantum estimation theory. The purpose of our specialized QEC is to preserve the QFI, which determines the best precision of estimating the value of a parameter, instead of the quantum states themselves. We have given testable conditions to identify the errors to which the QFI is immune, and constructed the optimal measurements in noisy states for the best estimation precision. While in the standard QEC any states, mixed or pure, in the coding subspace can be used in a metrological scheme, our conditions do not generally give rise to a subspace, instead only a special set of states that can serve our purpose. Our method can be readily applied for some parameter estimation problems, especially for those in the stabilizer formalism. Comparing with the standard stabilizer codes, our theory has the advantages of, firstly, being capable of preserving QFI against more errors using the same amount of resources and, secondly, sparing the recovery operations. Condition for preserving QFI Let us start with a crucial observation on the loss of QFI after a known noisy channel. For a given channel with Kraus operators { E j }, we denote V a unitary representation on the system plus an ancilla in the state ρ a such that where Tr a is the partial trace over the ancilla. For the sake of rigorousness, we assume that we always have bounded SLD operators henceforth, that is, SLD operators L θ and for states ρ θ and , respectively, exist and are finite. The loss of QFI can be expressed as (see Supplementary Note 1 ) where denotes the set of all bounded Hermitian operators on the Hilbert space associated with the output of , is the Hilbert–Schmidt norm of the operator O , and is exactly the square of the measurement error used by Ozawa to derive his error–disturbance uncertainty relation [46] . From equation (13), we see that the loss of QFI can be understood as the minimal measurement error of measuring a Hermitian operator Q after the given noisy channel compared with measuring L θ before the noisy channel. We note that due to equation (13), the following statements are equivalent: a . b There exists a Hermitian operator Q such that is satisfied for all j . c is satisfied for all j . Sketch of the proof The necessary and sufficient condition (4) for the preservation of QFI under a known noisy channel follows from the equivalence between (a) and (c). Theorem 1 is a consequence of equation (4). The geometric picture illustrated in Fig. 2 is due to the equivalence between (a) and (b). Theorem 2 is implied by the equivalence between (a) and (b) together with the following lemma, for which we give a constructive proof in Supplementary Note 1 . Lemma 1: for two indexed families of vectors | s j 〉 and | d j 〉, there exists a Hermitian operator Q such that Q | s j 〉=| d j 〉 for all j , if and only if (i) 〈 s j | d k 〉=〈 d j | s k 〉 for all j and k and (ii) for all a j such that , must be satisfied. Theorem 3 follows from the satisfaction of the two testable conditions in Theorem 2 for the errors with τ =0,1, where is a Pauli error that commutes with the stabilizer of the code S and anticommutes with Δ H eff . The full proof is presented in Supplementary Note 1 . The theorems and the lemma in this paper are also valid for infinite dimensional systems, as long as the SLD operator for the given parametric family of states is bounded. How to cite this article : Lu, X. M. et al . Robust quantum metrological schemes based on protection of quantum Fisher information. Nat. Commun. 6:7282 doi: 10.1038/ncomms8282 (2015).